Structure of the mammalian oligosaccharyl-transferase complex in the native ER protein translocon In mammalian cells, proteins are typically translocated across the endoplasmic reticulum (ER) membrane in a co-translational mode by the ER protein translocon, comprising the protein-conducting channel Sec61 and additional complexes involved in nascent chain processing and translocation. As an integral component of the translocon, the oligosaccharyl-transferase complex (OST) catalyses co-translational N-glycosylation, one of the most common protein modifications in eukaryotic cells. Here we use cryoelectron tomography, cryoelectron microscopy single-particle analysis and small interfering RNA-mediated gene silencing to determine the overall structure, oligomeric state and position of OST in the native ER protein translocon of mammalian cells in unprecedented detail. The observed positioning of OST in close proximity to Sec61 provides a basis for understanding how protein translocation into the ER and glycosylation of nascent proteins are structurally coupled. The overall spatial organization of the native translocon, as determined here, serves as a reliable framework for further hypothesis-driven studies. In mammalian cells, co-translational N-glycosylation is one of the most common covalent protein modifications. This essential reaction is catalysed by the oligosaccharyl-transferase complex (OST) [1] , [2] , [3] , an elaborate multisubunit complex integrated into the endoplasmic reticulum (ER) protein translocon. The catalytic OST subunit is present in two paralogous forms, STT3A and B, joined by at least six accessory subunits of poorly understood function: ribophorin I (RibI), ribophorin II (RibII), OST48, DAD1, N33 or IAP, and OST4. Sequence analysis and proteinase protection assays [4] suggest that all OST subunits are integral membrane proteins and many possess substantial lumenal domains, adding up to nearly 200 kDa [2] ( Supplementary Fig. 1 ). Despite its essential function, structural information on OST and its integration into the ER protein translocon is sparse and inconclusive. Recently, we gained first insights into the organization of the native translocon from a reconstruction of endogenous 80S ribosomes, attached to canine pancreatic rough microsomes (RMs), obtained using cryoelectron tomography (CET) and subtomogram analysis [5] . In the ribosome-associated density corresponding to the translocon, we discerned several membrane-embedded and lumenal complexes, including the protein-conducting channel Sec61, the translocon-associated protein complex (TRAP) and a large lumenal density, protruding 9 nm into the lumen. In this work, we localize OST in the native mammalian ER protein translocon using CET in combination with small interfering RNA (siRNA)-mediated gene silencing in human cells. Determining the structure of ribosome nascent chain complexes (RNCs) bound either to the native or solubilized translocon of canine pancreatic microsomes using CET and single-particle analysis (SPA) allows dissecting the structure and integration of OST in the mammalian translocon in unprecedented detail. Confirming the position of TRAP in the native translocon As a control for following silencing experiments, we first analysed RMs from HeLa cells that were treated with non-silencing siRNA. Classification of automatically located and iteratively aligned subtomograms depicting ER membrane-associated ribosomes revealed that two distinct populations of translocons were present in the data, including (42%) and lacking (58%) a large lumenal density (LD) ( Supplementary Fig. 2a ). For the final subtomogram average ( Fig. 1a ), only particles including LD were retained, yielding a resolution of 40 Å. The average shares all low-resolution features with the map of the canine ER-associated ribosome we previously reported [5] , and was used as a control map for the evaluation of different knockdown structures in the following. 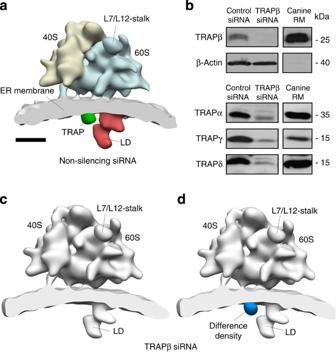Figure 1: Localization of TRAP in a subtomogram average of the human ER membrane-associated ribosome. (a) Subtomogram average for microsomes, isolated from HeLa cells treated with non-silencing control siRNA. Only particles including LD were retained for the average (Supplementary Fig. 2a). Scale bar, 10 nm. (b) HeLa cells were treated with TRAPβ or control siRNA. Protein levels of the target protein, as well as of TRAPα, γ and δ afterTRAPβgene silencing were analysed by SDS–PAGE and western blot analysis. As a positive control for the TRAP antibodies, an aliquot of rough canine microsomes (RMs) was run in parallel. The differences in intensity in the canine RMs compared with HeLa total lysate are due to the different concentrations of ER proteins in the samples and species differences in antibody affinity. (c,d) The subtomogram average for microsomes, isolated from TRAPβ-depleted HeLa cells is shown with (d) and without (c) the difference density to the control, isosurface rendered at 6σ(blue). All structures were filtered to a resolution of 40 Å. Figure 1: Localization of TRAP in a subtomogram average of the human ER membrane-associated ribosome. ( a ) Subtomogram average for microsomes, isolated from HeLa cells treated with non-silencing control siRNA. Only particles including LD were retained for the average ( Supplementary Fig. 2a ). Scale bar, 10 nm. ( b ) HeLa cells were treated with TRAPβ or control siRNA. Protein levels of the target protein, as well as of TRAPα, γ and δ after TRAPβ gene silencing were analysed by SDS–PAGE and western blot analysis. As a positive control for the TRAP antibodies, an aliquot of rough canine microsomes (RMs) was run in parallel. The differences in intensity in the canine RMs compared with HeLa total lysate are due to the different concentrations of ER proteins in the samples and species differences in antibody affinity. ( c , d ) The subtomogram average for microsomes, isolated from TRAPβ-depleted HeLa cells is shown with ( d ) and without ( c ) the difference density to the control, isosurface rendered at 6 σ (blue). All structures were filtered to a resolution of 40 Å. Full size image As a proof-of-principle for the gene-silencing approach, TRAPβ was chosen as a target due to the previously established position of TRAP in the detergent-extracted translocon by cryoelectron microscopy (cryo-EM) SPA [6] . TRAPβ ( SSR2 ) gene silencing for 96 h did not have major effects on cell growth (88±7% s.e.m. of control siRNA-treated cells; n =4), ER integrity ( Table 1 ), ER morphology ( Supplementary Fig. 3b ), protein translocation and substrate processing ( Supplementary Fig. 4a ). Western blotting indicates a nearly quantitative depletion of the target protein as well as all other TRAP subunits ( Fig. 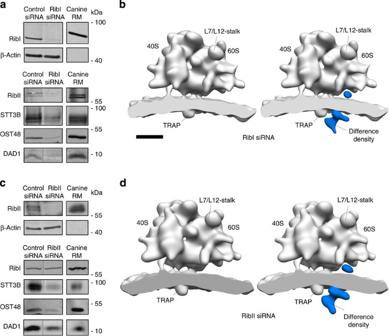Figure 2: Localization of OST in subtomogram averages of the human ER membrane-associated ribosome. HeLa cells were treated with RibI (a,b) or RibII (c,d) and control siRNA. Protein levels of the target proteins, as well as non-target OST subunits after RibI (a) or RibII (c) gene silencing were analysed by SDS–PAGE and western blot analysis. As a positive control for the OST antibodies, an aliquot of rough canine microsomes (RMs) was run in parallel. The differences in intensity in the canine RMs compared with HeLa total lysate are due to the different concentrations of ER proteins in the samples and species differences in antibody affinity. The subtomogram averages for microsomes, isolated from RibI- (b) or RibII- (d) depleted HeLa cells are shown with (right) and without (left) the difference density to the control, isosurface rendered at 6σ(blue). All structures were filtered to a resolution of 40 Å. Scale bar, 10 nm. 1b and Table 2 ), as previously observed [7] . As there was no decrease in the transcription of the TRAPα ( SSR1 ) gene ( Supplementary Fig. 5a ), depletion of non-target TRAP subunits was most likely to be due to destabilization of TRAP and subsequent degradation of subunits. Consistent with the control data set, translocons including (43%) and lacking (57%) LD were present in the TRAPβ knockdown data ( Supplementary Fig. 2b ). Again, only particles including LD were retained for the final average. Different from the control, essentially the entire density assigned to TRAP disappeared ( Fig. 1c ), which is also highly significant in the difference map to the control ( Fig. 1d ). Thus, the position of TRAP, previously assigned based on the purified and solubilized ribosome–Sec61–TRAP complex [6] , was confirmed in situ and we concluded that a 60-kDa lumenal density can be localized accurately using in situ CET in combination with gene silencing. Table 1 Relative protein content of selected ER-resident proteins after silencing with the indicated siRNA. Full size table Table 2 Relative protein content of TRAP and OST subunits after silencing with the indicated siRNA. Full size table Identification and localization of OST in the native translocon On the basis of its size and position close to Sec61, we speculated that LD might represent the nascent-chain-processing OST complex. Therefore, we depleted HeLa cells of either RibI or RibII, both integral OST subunits. Silencing of RPN1 and RPN2 , coding for RibI and RibII, respectively, for 72 h only had mild effects on cell growth (88±5% s.e.m. ( n =6) and 76±16% s.e.m. ( n =3) of control siRNA-treated cells for RibI and RibII, respectively), ER integrity ( Table 1 ), ER morphology ( Supplementary Fig. 3c,d ) and protein translocation activity ( Supplementary Fig. 4b ). For the RibI knockdown, western blotting indicates a strong reduction of the target protein (<10% residual protein) and also partial depletion of at least four other OST subunits (RibII, STT3B, OST48 and DAD1; Fig. 2a and Table 2 ), analogous to knockdown studies of other OST subunits [8] . For the RibII knockdown, nearly quantitative depletion of the target protein and strong reduction of three out of the four other OST subunits (STT3B, OST48 and DAD1) was observed, whereas RibI was only moderately affected ( Fig. 2c and Table 2 ). Reverse transcription–PCR (RT–PCR) data indicate that depletion of non-target OST subunits is due to protein degradation for both knockdowns ( Supplementary Fig. 5b,c ). As reported previously [9] , depletion of RibI resulted in only a mild and selective glycosylation defect ( Supplementary Fig. 4b ). We suggest that single catalytically active STT3 subunits may be able to independently perform N-glycosylation after RibI depletion. The subtomogram averages of both knockdown samples and their difference maps to the control are largely identical ( Fig. 2b,d ): essentially all density assigned to LD in the control map disappeared, confirming our hypothesis that LD represents or at least includes OST. A second, significant reduction of density in the knockdowns can be observed at the cytosolic face of the ER membrane, directly opposed to LD. This density may correspond to cytosolic domains of OST and possibly associated proteins. Figure 2: Localization of OST in subtomogram averages of the human ER membrane-associated ribosome. HeLa cells were treated with RibI ( a , b ) or RibII ( c , d ) and control siRNA. Protein levels of the target proteins, as well as non-target OST subunits after RibI ( a ) or RibII ( c ) gene silencing were analysed by SDS–PAGE and western blot analysis. As a positive control for the OST antibodies, an aliquot of rough canine microsomes (RMs) was run in parallel. The differences in intensity in the canine RMs compared with HeLa total lysate are due to the different concentrations of ER proteins in the samples and species differences in antibody affinity. The subtomogram averages for microsomes, isolated from RibI- ( b ) or RibII- ( d ) depleted HeLa cells are shown with (right) and without (left) the difference density to the control, isosurface rendered at 6 σ (blue). All structures were filtered to a resolution of 40 Å. Scale bar, 10 nm. Full size image The only further known component of the translocon that contains notable lumenal segments (47 kDa) is the signal peptidase complex (SPase) [10] . To rule out the possibility that LD corresponds to an OST–SPase supercomplex, we also depleted SPase subunits from HeLa cells and analysed the derived microsomes by CET. Comparison with the control structure revealed no significant reduction of density in the resulting subtomogram average ( Supplementary Fig. 6 ). Consistent with CET analysis of the SPase knockdown, depletion of OST subunits did not affect the stability of SPase subunits, as judged by western blotting ( Table 1 ). In conclusion, LD does not comprise SPase and thus most probably corresponds to OST alone. This positioning of OST in the native translocon allows for concomitant scanning of a nascent polypeptide for glycosylation sites, while it is conducted into the ER lumen, thus providing a basic understanding of how protein translocation into the ER and glycosylation of nascent proteins are structurally coupled. From the good agreement of the approximate molecular weight of LD (170–200 kDa) with the lumenal mass of OST, as well as the absence of multiply-occurring structural features in LD, we furthermore conclude that OST is present in only one copy in the native translocon, in contrast to previous hypotheses of a dimeric OST organization [11] . Structure and integration of OST in the native translocon To resolve native OST and its surroundings at a greater level of detail, we used a cell-free translation/translocation system to populate vacant translocons of ribosome-stripped canine pancreatic microsomes with homogenous RNCs stalled on the regulatory peptide of the human cytomegalovirus (CMV) gp48 upstream open-reading frame 2 (ref. 12 ). Quantitative stalling and high translocation efficiency (~95%) in the cell-free system were verified by SDS–polyacrylamide gel electrophoresis (SDS–PAGE) and western blotting ( Supplementary Fig. 7 ). ER membrane-associated ribosomes from tomographic reconstructions ( Supplementary Fig. 8 ) were iteratively aligned and classified, confirming the presence of two distinct populations of translocons, including (63%) and lacking (37%) OST ( Supplementary Fig. 2e ). The ribosome bound to the OST-containing translocon ( Fig. 3a ) was resolved to 22 Å ( Supplementary Figs 9 and 10 ) and shares all low-resolution features with the endogenous human ER membrane-associated ribosome ( Fig. 1a ). The translocon is embedded into a well-resolved membrane bilayer and dense regions that transverse the membrane can be distinguished ( Fig. 3b–e ), likely to be corresponding to tightly packed transmembrane segments of integral membrane proteins, referred to as membrane anchors (MAs) in the following. In the density, the hook-shaped lumenal part of OST is connected to the ER membrane by two MAs ( Fig. 3d,e ), one of them likely to be corresponding to the tightly packed 13-transmembrane helices of the catalytic subunit STT3 (ref. 13 ). 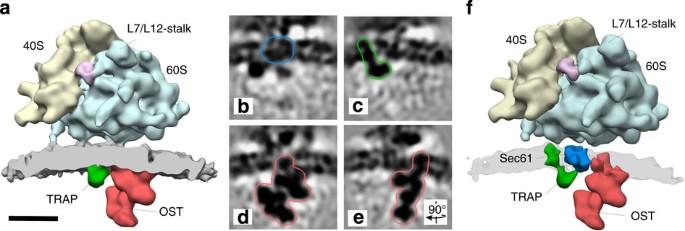Figure 3: Subtomogram average of the stalled mammalian ribosome bound to canine pancreatic microsomes. (a) Subtomogram average at 22 Å resolution. On the ribosomal stalk base, additional non-ribosomal density is resolved (magenta) that potentially corresponds to canonical translation, elongation or termination factors. Scale bar, 10 nm. (b–e) Structural details of the membrane and ER lumenal region of the subtomogram average after alignment focused on this region. Lumenal and/or transmembrane segments (outlined) of Sec61 (b) (as identified inSupplementary Fig. 11), TRAP (c) and OST (d,e) can be discerned. Slices inb–dare oriented as inf, the slice ineis rotated by 90°. (f) Lumenal and transmembrane segments of OST (red), Sec61 (dark blue) and TRAP (green) were automatically segmented from the subtomogram average. Figure 3: Subtomogram average of the stalled mammalian ribosome bound to canine pancreatic microsomes. ( a ) Subtomogram average at 22 Å resolution. On the ribosomal stalk base, additional non-ribosomal density is resolved (magenta) that potentially corresponds to canonical translation, elongation or termination factors. Scale bar, 10 nm. ( b – e ) Structural details of the membrane and ER lumenal region of the subtomogram average after alignment focused on this region. Lumenal and/or transmembrane segments (outlined) of Sec61 ( b ) (as identified in Supplementary Fig. 11 ), TRAP ( c ) and OST ( d , e ) can be discerned. Slices in b – d are oriented as in f , the slice in e is rotated by 90°. ( f ) Lumenal and transmembrane segments of OST (red), Sec61 (dark blue) and TRAP (green) were automatically segmented from the subtomogram average. Full size image To locate the Sec61 protein-conducting channel in the subtomogram average, a single-particle reconstruction of the canine ribosome (EMD 1480) [14] and an aligned atomic model of the nascent-chain-translocating canine Sec61 complex [15] were fitted into the subtomogram average as one rigid body. Near the ribosomal tunnel exit, a high-density region of the subtomogram average ( Fig. 3b ) exactly co-localizes with the fitted atomic model of Sec61 ( Supplementary Fig. 11 ), allowing an unambiguous identification of Sec61 in the translocon density. Directly adjacent to the density attributed to Sec61, TRAP is resolved with its prominent ER-lumenal domain and one MA ( Fig. 4c ). 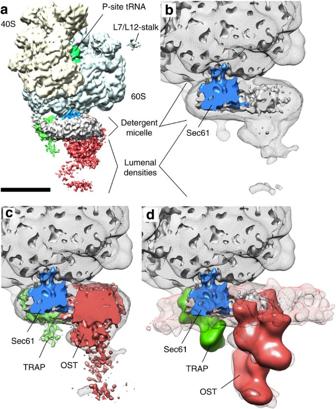Figure 4: Single-particle reconstruction of stalled ribosomes bound to solubilized canine Sec61–OST–TRAP complexes. (a) Reconstruction filtered to 10 Å resolution. Colouring as inFig. 3f. Scale bar, 10 nm. (b) Magnified view of the reconstruction with Sec61 segmented from the map (blue). The overall density is shown at two different resolutions and threshold levels (grey) to visualize the high-resolution details of Sec61, but also the overall structure of the translocon. (c,d) Additional densities in the single-particle reconstruction (c) co-localize with the isolated TRAP and OST densities from the subtomogram average (d). Figure 4: Single-particle reconstruction of stalled ribosomes bound to solubilized canine Sec61–OST–TRAP complexes. ( a ) Reconstruction filtered to 10 Å resolution. Colouring as in Fig. 3f . Scale bar, 10 nm. ( b ) Magnified view of the reconstruction with Sec61 segmented from the map (blue). The overall density is shown at two different resolutions and threshold levels (grey) to visualize the high-resolution details of Sec61, but also the overall structure of the translocon. ( c , d ) Additional densities in the single-particle reconstruction ( c ) co-localize with the isolated TRAP and OST densities from the subtomogram average ( d ). Full size image To visualize their spatial organization in the native translocon, lumenal and transmembrane segments of OST, Sec61 and TRAP were automatically segmented from the subtomogram average ( Fig. 3f and Supplementary Movie 1 ), revealing a potential interface between Sec61 and OST within the ER membrane ( Supplementary Fig. 12 ). To analyse this interaction in more detail, we compared the subtomogram average to a reconstruction by cryo-EM SPA of wheatgerm RNCs bound to the mammalian translocon. Although detergent solubilization yielded primarily RNC–Sec61 complexes [15] , particle sorting also revealed an additional less-populated class that is similar to the subtomogram average ( Fig. 4a ). It is known that TRAP and OST co-purify under mild solubilization conditions with Sec61 as part of the so-called RAMP fraction (ribosome-associated membrane proteins) [16] , and mass spectrometry (MS) analysis indeed confirmed that among the 100 most abundant proteins in the sample, there are almost exclusively ribosomal proteins and subunits of the Sec61, TRAP and OST complexes ( Supplementary Data 1 ). Therefore, the observed similarity strongly suggests that this particle population corresponds to RNCs bound to the Sec61–OST–TRAP complex. The local resolution of Sec61 is in the range of the global resolution of the single-particle reconstruction (10 Å), but TRAP and OST are less well resolved, probably due to underrepresentation or a higher degree of flexibility in the detergent micelle. Secondary structure elements of Sec61 that are resolved in several areas of the map ( Fig. 4b and Supplementary Fig. 13 ) allowed us to accurately position the protein-conducting channel in the translocon and to fit an atomic model of the nascent-chain-translocating heterotrimeric Sec61 complex ( Supplementary Fig. 13 ) [15] . Notably, the position and overall arrangement of the Sec61 complex in the presence of TRAP and OST remain indistinguishable from the canonical position observed previously for the ribosome-bound Sec61 or SecYEG complexes alone [17] , [18] . Superposition of the subtomogram average and the single-particle reconstruction showed a spatial coincidence of the translocon densities ( Fig. 4c,d ) and allowed accurate positioning of Sec61 in relation to OST and TRAP in the subtomogram average. Here, one of the two MAs of OST is in direct proximity to the carboxy-terminal region of Sec61γ and a hinge helix between the amino- and the C-terminal halves of Sec61α ( Fig. 5 and Supplementary Fig. 13 ), suggesting that this interface contributes to the stable integration of OST into the translocon. 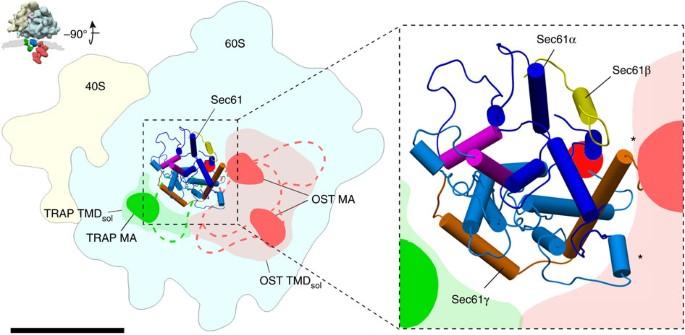Figure 5: Spatial organization of OST, Sec61 and TRAP in the translocon seen from the ER lumen. For TRAP (green) and OST (red), MAs and lumenal segments (dashed lines) from the native translocon, as well as transmembrane density from the solubilized translocon (TMDsol) were projected onto the membrane plane. Atomic models for Sec61α (N-terminal half: dark blue; C-terminal half: light blue), Sec61β (yellow) and Sec61γ (orange), as well as the position of the peptide exit tunnel (red dot) on the large ribosomal subunit and the Sec61 lateral gate (magenta helices), are depicted. One of the two MAs of OST is in proximity to the C-terminal region of Sec61γ and a hinge helix between the N- and the C-terminal halves of Sec61α (asterisks). Scale bar, 10 nm. Figure 5: Spatial organization of OST, Sec61 and TRAP in the translocon seen from the ER lumen. For TRAP (green) and OST (red), MAs and lumenal segments (dashed lines) from the native translocon, as well as transmembrane density from the solubilized translocon (TMD sol ) were projected onto the membrane plane. Atomic models for Sec61α (N-terminal half: dark blue; C-terminal half: light blue), Sec61β (yellow) and Sec61γ (orange), as well as the position of the peptide exit tunnel (red dot) on the large ribosomal subunit and the Sec61 lateral gate (magenta helices), are depicted. One of the two MAs of OST is in proximity to the C-terminal region of Sec61γ and a hinge helix between the N- and the C-terminal halves of Sec61α (asterisks). Scale bar, 10 nm. Full size image In this work, we used CET, SPA and siRNA-mediated gene silencing to determine the overall structure, oligomeric state and position of OST in the native ER protein translocon of mammalian cells. The position of OST in close proximity to Sec61 ( Fig. 5 ) agrees well with crosslinking studies, indicating proximity of OST to both the large ribosomal subunit [19] and the Sec61 complex [20] , and it is also consistent with negative-stain EM images of ribosomal particles, showing additional density close to the ribosomal tunnel exit on complex formation with OST [21] . In the overall arrangement of the translocon determined here ( Fig. 5 ), the directly adjacent OST and TRAP complexes spatially confine the C-terminal segment of Sec61α. This is in agreement with a rigid positioning of the C-terminal half of Sec61 on the ribosome in different functional states [15] . The N-terminal segment of Sec61α, in contrast, is spatially less constrained, which may be required to adopt the observed more open states during peptide translocation or membrane insertion [15] . Notably, the Sec61 lateral gate, through which transmembrane helices of nascent membrane proteins are released into the membrane bilayer, points away from OST ( Fig. 5 ). The resulting distant positioning of OST from nascent transmembrane helices may explain why glycosylation consensus motifs have to be located more than 12–15 amino acid residues (~3–5 nm) away from a transmembrane helix to be glycosylated efficiently during translocation into the ER lumen [22] . In contrast to the excellent agreement of the position of OST in the native translocon determined here with previously established biochemical information, the structure of native mammalian OST itself ( Fig. 3 ) is difficult to reconcile with a previous single-particle study of detergent-solubilized, isolated yeast OST [23] . In the latter reconstruction, the overall shape of OST appears much more compact than determined here, while the surface appears unusually ragged. The structural discrepancy between the native mammalian OST structure and the single-particle reconstruction of detergent-solubilized, isolated yeast OST may be due to interspecies differences in the size of the RibI and RibII subunits, different conformational states of the complex, destabilization of OST in the detergent micelle, or the high error margin in cryo-EM single-particle reconstructions of small detergent-extracted complexes. Cryo-EM single-particle reconstructions can bear significant errors, as recently discussed [24] , [25] . This holds true in particular for detergent-extracted complexes, because the particles tend to be heterogeneous due to the formation of micelles, and for small complexes (traditionally below ~300–500 kDa), because the amount of signal may be insufficient for accurate alignment of the single particles [26] . An unexpected finding in our analysis of the translocon is that in all microsome data sets analysed in this work, two distinct translocon populations—including and lacking OST—were present (excluding the RibI and RibII knockdown tomograms, of course; Supplementary Figs 2 and 6 ). Albeit it cannot be entirely ruled out that partial dissociation of OST is induced by microsome formation at this point, the fact that OST remains partially associated to Sec61 even after detergent solubilization, and the tight interaction between Sec61 and OST observed in our subtomogram average, both suggest that translocon populations including and lacking OST also coexist in the cell. Whether OST is recruited transiently to the translocon during translocation of nascent peptides or whether two stable, specialized species of translocon complexes exist and how co-translational glycosylation of nascent peptides is assured remains subject to future studies. In summary, the spatial organization of the translocon described here provides a basis for understanding how protein translocation into the ER and N-glycosylation of nascent proteins are structurally coupled and it serves as a reliable framework for further hypothesis-driven functional studies. In conjunction with orthogonal structural data, our density of the translocon may also allow dissecting the TRAP and OST complexes in further detail using integrative approaches in the future [27] . Cell culture HeLa cells (ATCC number CCL-2) were cultured in DMEM (Gibco-Invitrogen, Karlsruhe, Germany) containing 10% FBS (Biochrom, Berlin, Germany) and 1% penicillin and streptomycin (PAA, Pasching, Austria) in a humidified environment with 5% CO 2 at 37 °C. Gene silencing of HeLa cells For gene-silencing experiments, 1.2 × 10 6 HeLa cells were seeded per 10-cm culture dish and transfected with RibI siRNA (5′-CGU ACA UUG AGA AUG AGA AdTdT-3′; Qiagen, Hilden, Germany) for silencing of RPN1 gene, RibII siRNA (5′-GGC UAU CUU GCG GUU GCA AdTdT-3′; Qiagen) for silencing of RPN2 gene or SPC25 siRNA (5′-CCA UGA CAG UCU UGC CAU AdTdT-3′; Qiagen) for silencing of SPC25 gene, respectively, at a final concentration of 25 nM using HiPerFect Reagent (Qiagen). After 24 h, the medium was changed and the cells were transfected a second time. SSR2 gene silencing was carried out according to the same protocol with TRAPβ siRNA (5′-AAG GGU AUC UUA AAU GCA AdTdT-3′; Qiagen) at a final concentration of 10 nM. The non-silencing AllStars Negative Control siRNA (Qiagen) served as control siRNA. Silencing was evaluated by RT–PCR and western blot analysis as described. Quantitative RT–PCR analysis Cells were harvested and total RNA was isolated using the QIAamp RNA Blood Kit (Qiagen). Reverse transcription of mRNA was performed with Superscript II RT (Invitrogen, Darmstadt, Germany) and oligo(dT) primers (Invitrogen), and the resulting complementary DNA was purified using the PCR Purification Kit (Qiagen). TaqMan Gene Expression Assays (Applied Biosystems, Darmstadt, Germany) were used for quantitative real-time RT–PCR of TRAPα (Hs00162340_m1), TRAPβ (Hs00162346_m1), RPN1 (Hs00161446_m1), RPN2 (Hs00955802_m1), STT3B (Hs00385811_m1), DDOST (Hs00193263_m1) and DAD1 (Hs02912874_m1) in a StepOne Plus 96-well system (Applied Biosystems). Relative gene expression was calculated using the comparative C T method [28] with ACTB (Hs00357333_g1) serving as internal control. ΔCt values were then normalized to control siRNA-treated cells. Semi-quantitative western blot analysis Rabbit antibodies were raised against the C-terminal peptides of human Sec61α (14-mer), SPase22/23 (14-mer), SPase25 (11-mer), Sec62 (11-mer) and TRAPα (15-mer), or the N-terminal peptides of human BiP (12-mer), human SPase12 (15-mer) and Grp170 (11-mer) plus an N- or C-terminal cysteine, human TRAPβ (aa 18–32) and human SRα (aa 137–150), plus a C-terminal cysteine, dog GRP94, human Sec63-ΔN380 and murine ERj1C-ΔN21 (ref. 29 ). Antibodies directed against RibI, RibII, STT3B and DAD1 were a kind gift from S. High (Manchester, UK). The ERp57 antibody was a kind gift from T. Wileman (Norwich, UK). Antibodies directed against OST48 (Santa Cruz Biotechnology, Heidelberg, Germany), Calnexin (Stressgene, Hamburg, Germany) and TRAPγ, TRAPδ and β-actin (Sigma, Taufkirchen, Germany) were obtained from commercial sources. The primary antibodies were visualized using peroxidase-conjugated anti-rabbit IgG-goat antibodies (Sigma), ECL Plex goat anti-rabbit IgG-Cy5 conjugate or ECL Plex goat anti-mouse IgG-Cy3 conjugate (GE Healthcare, Freiburg, Germany) and X-ray films (GE Healthcare), or the Typhoon-Trio imaging system (GE Healthcare) in combination with Image Quant TL software 7.0 (GE Healthcare). Full scans of all western blottings are shown in Supplementary Figs 14–18 . Working dilutions of all antibodies and catalogue numbers of purchased antibodies are listed in Supplementary Table 1 . Protein transport assays Precursor polypeptides were synthesized in reticulocyte lysate (nuclease treated; Promega, Heidelberg, Germany) in the presence of [ 35 S]methionine (Perkin Elmer, Rodgau-Jügesheim, Germany) plus buffer or semipermeabilized cells for 60 min at 30 °C. Semipermeabilized cells were prepared from identical cell numbers according to a published procedure [30] . All samples were analysed by SDS–PAGE and phosphorimaging using the Typhoon-Trio imaging system (GE Healthcare) in combination with Image Quant TL software 7.0 (GE Healthcare). Full phosphorimaging scans are shown in Supplementary Fig. 19 . Immunofluorescence microscopy Cells were fixed with paraformaldehyde, washed and an indirect immunofluorescence staining was performed with an affinity-purified rabbit anti-peptide antibody directed against the human Sec62 (C-terminal 11-mer plus an N-terminal cysteine) and Alexa-Fluor-594-coupled secondary antibody from goat (Invitrogen). We note that the anti-Sec62 antibody is specific for Sec62 under denaturing as well as native conditions (that is, western blotting and fluorescence microscopy signals were quenched after silencing of the SEC62 gene) [31] . Cells were analysed by microscopy using an Elyra SIM (Carl Zeiss MicroImaging, Göttingen, Germany). Synthesis of the Sec62 protein was not affected by RPN1 , RPN2 and TRAPβ gene silencing ( Table 1 ). Preparation of RMs from culture cells siRNA-treated cells (30 × 10 6 ) were harvested and washed once with PBS and twice with HEPES buffer (50 mM HEPES/KOH, pH 7.5; 0.25 M sucrose; 50 mM KOAc; 6 mM MgOAc; 4 mM phenylmethylsulphonyl fluoride; 1 mM EDTA; 1 mM dithiothreitol (DTT); 0.1 mg ml −1 cycloheximide; 0.3 U ml −1 RNAsin (Promega, Heidelberg, Germany); protease inhibitor cocktail). After homogenization using a glass/Teflon homogenizer, the suspension was centrifuged at 1,000 g for 10 min. The supernatant was centrifuged at 10,000 g for 10 min. The new supernatant was layered onto a 0.6-M sucrose cushion (50 mM HEPES/KOH, pH 7.5; 0.6 M sucrose; 100 mM KOAc; 5 mM MgOAc; 4 mM DTT; 0.1 mg ml −1 cycloheximide; 40 U ml −1 RNAsin) and centrifuged at 230,000 g for 90 min. The resulting membrane pellet was resuspended in HEPES buffer and stored at −80 °C. All steps after the first washing step were carried out on ice. Preparation of stripped canine pancreatic RMs RMs were prepared from dog pancreas as previously described [5] . RMs in buffer A (20 mM Hepes, pH 7.6; 50 mM KCl; 2 mM MgCl 2 ; 200 mM sucrose; 2 mM DTT; protease inhibitor) were incubated for 30 min at 20 °C in the presence of 0.5 mM GTP (Sigma-Aldrich, Germany), 2 mM puromycin (Sigma-Aldrich), 750 mM KOAC (Sigma-Aldrich) and subsequently pelleted (TLA 100 rotor, 160,000 g , 35 min, 20 °C). The microsomal pellet was resuspended in buffer B (50 mM HEPES, pH 7.6; 1.25 M sucrose; 800 mM CsCl; 15 mM Mg(OAc) 2 ; 3 mM DTT; protease inhibitor) and layered on the bottom of a two-step gradient consisting of buffer C (buffer B, only 0.8 M sucrose) and buffer A. After flotation (TLA 120.2 rotor, 350,000 g , 70 min, 20 °C), microsomes could be retrieved from the interphase between buffer A and C. Ribosome-stripped microsomes were pelleted (TLA 100 rotor, 160,000 g , 35 min, 4 °C), resuspended in buffer A at a concentration of 1 eq μl −1 , flash frozen in liquid nitrogen and stored at −80 °C. Cell-free system for CET The pre-pro-lactin (ppl) construct with C-terminal CMV stalling sequence (ppl-CMV) was generated using a primer extension PCR reaction based on the pB4 plasmid [32] with forward primer 5′-TAT TTA GGT GAC ACT ATA GAA GAG GCC GCC ACC ATG GAC AGC AAA GGT TCG TC-3′ and reverse primer 5′-TTA AGG AGG AAT ATA TTT GCA GGT CAG CAG GCT GCT CAG TTT TTT CGC ACT CAG CAC CAG CGG TTC CAT GCA GTT GTT GTT GTA GAT GAT TCT G-3′. Stalling ppl-CMV mRNA was prepared in vitro (mmessage mmachine SP6 Kit, Ambion, USA). Cell-free reactions were performed at 30 °C in Flexi rabbit reticulocyte lysate (Promega, USA) in the presence of 1 mM biotinylated Lysyl-transfer RNA (Transcend tRNA Kit, Promega, USA). Reactions were supplemented with 200 nM of non-stalling ppl or stalling ppl-CMV mRNA and puromycin/high-salt-treated rough membrane (PK-RM) at a concentration of 4 eq per 25 μl, where indicated. After 20 min, reactions were stopped on ice. For RNAse digestion assays, 20 μl of cell-free reaction were supplemented with 0.1 mg ml −1 (f.c.) RNAse A (Sigma-Aldrich, Germany) and incubated for 30 min at 30 °C. Ribosome association of ppl-CMV chains was analysed by pelleting ribosomes from 20 μl of cell-free reaction (without PK-RM) through a 0.25 M sucrose cushion (TLA 100, 30 min, 150,000 g , 4 °C). Translocation of ppl-CMV nascent chains was analysed by pelleting microsomes from 20 μl of cell-free reaction (eppendorf Centrifuge 5417R, 3 min, 16,000 g , 4 °C). Samples were analysed by SDS–PAGE and western blotting using streptavidin-coupled horseradish peroxidase (Transcend tRNA Kit, Promega, USA). Relative amounts of protein were quantified using AIDA two-dimensional densiometry software (Raytest, Germany). Cryoelectron tomography Twenty-five microlitres of in vitro reaction were centrifuged in an eppendorf Centrifuge 5417R (3 min, 16,000 g , 4 °C) to pellet microsomes. The pellet was resuspended in 25 μl of ribosome buffer (20 mM Hepes, pH 7.6; 50 mM KCl; 2 mM MgCl 2 ) and 3 μl were applied to lacey carbon molybdenum grids (Ted Pella, USA). After an incubation time of 60 s, 3 μl of 10-nm colloidal gold in ribosome buffer were added to the grid and the sample was vitrified in liquid ethane using a Vitrobot Mark IV (FEI Company, The Netherlands). Tilt series were acquired using a FEI Titan Krios TEM equipped with a 4k × 4k FEI Falcon direct electron detector. The TEM was operated at an acceleration voltage of 300 kV. Single-axis tilt series were recorded from −60° to +60° with an angular increment of 3° at a nominal defocus of 4 (canine pancreatic microsomes) or 8 μm (HeLa cell microsomes), and an object pixel size of 0.288 nm using the FEI tomography acquisition software. The cumulative electron dose did not exceed 60 electrons per Å 2 . Image processing for CET Phase correction of the tilt series, tomogram reconstruction (object pixel: 2.30 nm) and template matching (object pixel: 2.30 nm) were performed as described [5] . For tomograms obtained from canine pancreatic microsomes, subtomograms (32 3 voxels, object pixel: 2.30 nm) centred at the coordinates of the 1,000 highest-scoring peaks of the cross correlation function were classified using constrained principal component analysis [33] focusing on the large ribosomal subunit and the ER membrane. Classification separated ER membrane-associated ribosomes from most false-positive matches, such as gold markers, ER membrane or carbon edges. For tomograms obtained from HeLa cell microsomes, cross correlation peaks in areas containing rough ER were visually inspected to identify true-positive matches. For the selected coordinates, unbinned subtomograms (200 3 voxels, object pixel: 0.288 nm) were reconstructed individually from the weighted backprojections and aligned to the template using PyTom [34] . With a second round of constrained principal component analysis, translocons including and lacking the OST complex were sorted. Using aligned coordinates and angles, the reconstruction centre was moved to the centre of the translocon and unbinned subtomograms (96 3 voxels, object pixel: 2.88 Å) were reconstructed and aligned. The resolution of the resulting averages was determined by Fourier shell correlation (FSC) on appropriately masked averages (FSC=0.5) and cross resolution (FSC=0.33). We performed an independent reference-free alignment described in ref. 35 to rule out reference bias in the alignment process. This alternative alignment procedure divided the data into two halves that were aligned independently and assessed by FSC, commonly referred to as ‘gold standard FSC’ [36] . Normalized electron-density difference maps were generated from normalized tomographic reconstructions, filtered to their respective resolution. EM map analysis For EM map analysis, fitting of atomic models, segmentation and visualization, we used the UCSF Chimera software package [37] . Colouration of the EM maps was done either on single images in Photoshop by applying coloured layers (‘multiply’ style) to the image or in chimera on segmented densities. Sample preparation and data processing for SPA Bona fide translocating ribosome–Sec61 complexes were obtained using constructs based on the well-characterized Lep93 (here referred to as LepT) by Saaf et al. [38] These constructs contain glycosylation sites to precisely monitor the translocation state. We modified these constructs to generate and stabilize translocation and insertion intermediates by introducing a C-terminal ribosomal stalling sequence (CMV gp48 upstream open-reading frame) [12] , a streptavidin tag for affinity purification and an haemagglutinin tag for immunodetection. LepT-mRNA was used in a self-made wheatgerm translation system in the presence of PK-RM and signal recognition particle from dog pancreas [15] . After in vitro translation, ribosome-bound membranes were isolated and solubilized with digitonin. Programmed ribosomes containing the glycosylated LepT-peptide engaged with Sec61, OST and TRAP were affinity purified using the Strep-tag. For sample preparation, freshly prepared samples were applied to Quantifoil grids precoated with 2 nm carbon on top and flash frozen using the Vitrobot Mark IV (FEI Company). Data were collected on a Titan Krios TEM (FEI Company) under low-dose conditions at 200 keV and magnification of × 148,721 at the plane of the charge-coupled device using a TemCam-F416 CMOS camera (TVIPS GmbH), resulting in an image pixel size of 1.049 Å per pixel on the object scale. EM-TOOLS software was used for automated data collection and data were recorded in a defocus range of 1.3–4.0 μm. SPA and three-dimensional reconstruction was performed using the SPIDER software package [39] . Automated particle selection was performed using the programme Signature [40] , which was followed by a second automated particle classification step using the MAPPOS software [41] . Particles (487,470) were sorted for the presence of Sec61 complex and P-site tRNA, and remaining ‘non-particles’ representing noisy images or aggregated particles, which could not be excluded before. For sorting, in brief, references representing an empty ribosome, a programmed ribosome and a programmed ribosome bound to Sec61 were offered as references for supervised classification. ‘Non-particles’ were sorted out using a reference map derived from noise particles. After sorting, three-dimensional maps were obtained for a data subset (53,248 particles; 10.92%) containing highly enriched peptidyl–tRNA and Sec61 complex. From this data subset, a further subpopulation of 15,705 particles could be isolated, which contained a density larger than the Sec61 complex at the exit site. By MS analysis of the sample, the additional density was identified as the OST and TRAP complexes ( Supplementary Data 1 ). The RNC–Sec61–OST–TRAP data set could be refined to a global resolution of 9.3 Å, although the densities for TRAP and OST are not as well resolved. Accession codes: Subtomogram averages of the ER membrane-associated ribosome have been deposited in the EMDataBank with accession codes EMD- 2514 (silencing control), EMD- 2515 (TRAPβ knockdown), EMD- 2516 (RibI knockdown), EMD- 2517 (RibII knockdown), EMD- 2518 (SPC25 knockdown) and EMD- 2519 (stalled in cell-free system). The single-particle reconstruction of the stalled wheatgerm ribosome in complex with solubilized Sec61–TRAP–OST has been deposited with accession code EMD- 2523 . How to cite this article: Pfeffer, S. et al. Structure of the mammalian oligosaccharyl-transferase complex in the native ER protein translocon. Nat. Commun. 5:3072 doi: 10.1038/ncomms4072 (2014).